Precision spectroscopy by photon-recoil signal amplification Precision spectroscopy of atomic and molecular ions offers a window to new physics, but is typically limited to species with a cycling transition for laser cooling and detection. Quantum logic spectroscopy has overcome this limitation for species with long-lived excited states. Here we extend quantum logic spectroscopy to fast, dipole-allowed transitions and apply it to perform an absolute frequency measurement. We detect the absorption of photons by the spectroscopically investigated ion through the photon recoil imparted on a co-trapped ion of a different species, on which we can perform efficient quantum logic detection techniques. This amplifies the recoil signal from a few absorbed photons to thousands of fluorescence photons. We resolve the line centre of a dipole-allowed transition in 40 Ca + to 1/300 of its observed linewidth, rendering this measurement one of the most accurate of a broad transition. The simplicity and versatility of this approach enables spectroscopy of many previously inaccessible species. Precision optical spectroscopy of broad transitions provides information on the structure of molecules [1] , it allows tests of quantum electrodynamics [2] , and, through comparison with astrophysical data, probes for a possible variation of fundamental constants over cosmological scales [3] , [4] . Nuclear properties are revealed through isotope shift measurements [5] , [6] , [7] , [8] , [9] , or absolute frequency measurements [10] , [11] . Trapped ions are particularly well suited for such high precision experiments. The ions are stored in an almost field-free environment and can be laser-cooled to eliminate Doppler shifts. These features have enabled record accuracies in optical clocks [12] , [13] , [14] , [15] . For long-lived excited states such as in atoms with clock transitions, the electron-shelving technique amplifies the signal from a single absorbed photon by scattering many photons on a closed transition through selective optical coupling of one of the two spectroscopy states to a third electronic level [16] . The invention of quantum logic spectroscopy (QLS) [12] , [17] removed the need to detect the signal on the spectroscopically investigated ion (spectroscopy ion) by transferring the internal state information through a series of laser pulses to the co-trapped, so-called logic ion where the signal is observed via the electron-shelving technique. However, this original implementation of QLS requires long-lived spectroscopy states to implement the transfer sequence. For transitions with a short-lived excited state, spectroscopy of trapped ions is typically implemented through detection of scattered photons in laser-induced fluorescence [7] , [18] , [19] , [20] , [21] , [22] or detection of absorbed photons in laser absorption spectroscopy [23] . Neither of the two techniques reaches the fundamental quantum projection noise limit as in the electron-shelving technique [24] due to low light collection efficiency in laser-induced fluorescence and small atom-light coupling in laser absorption spectroscopy. In a variation of absorption spectroscopy, the detuning-dependent effect of spontaneous light forces on the motional state of trapped ions is employed to obtain a spectroscopy signal. This has been investigated by observing macroscopic heating on a Doppler-cooled two-ion crystal [25] , and through a measurement of motional phase change due to photon scattering [26] . Here, we present and demonstrate an extension of QLS, which combines the advantages of these techniques and provides a highly sensitive, quantum projection noise-limited signal for the spectroscopy of broad transitions. It is based on detection of momentum kicks from a few absorbed photons near the resonance of a single spectroscopy ion through a co-trapped logic ion. We demonstrate photon recoil spectroscopy (PRS) on the 2 S 1/2 ↔ 2 P 1/2 transition in a 40 Ca + ion, resolving the line by a factor of 1/300 of its observed linewidth of ~34 MHz and achieve a statistics-limited fractional instability of σ y ( τ )=5.1 × 10 −9 , corresponding to 100 absorbed photons for a resolution of 7.2 MHz. This proof-of-principle experiment demonstrates the potential of PRS and its applicability to different species. Spectroscopy scheme The principle of PRS is shown in Fig. 1 . Starting from the axial motional ground state of the two-ion crystal ( Fig. 1a ), momentum transfer from photon absorption on the spectroscopy ion results in motional excitation ( Fig. 1b ). Owing to the strong Coulomb interaction, this excitation is shared by the logic ion where it is converted into a long-lived internal excitation by applying a so-called red-sideband laser pulse, which changes the internal state conditioned on the presence of motional excitation ( Fig. 1c ) [27] , [28] , [29] . Subsequent electron-shelving detection on the logic ion amplifies the signal of a few absorbed photons on the spectroscopy ion to thousands of scattered photons on the logic ion, providing quantum projection noise-limited detection of motional excitation. This signal is background-free, since spectroscopy and detection are separated in time. 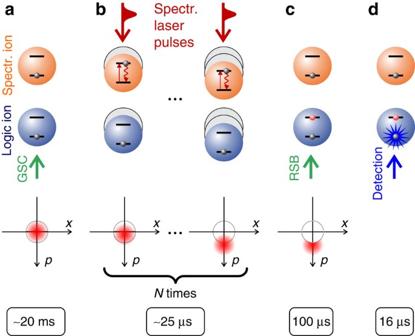Figure 1: Principle of PRS. The top part of the figure shows the internal and motional excitation of the two-ion crystal (spectroscopy (spectr.) ion: top, logic ion: bottom). The centre part shows the Wigner phase-space representation of the excited normal mode. Typical timescales for the experimental implementation are shown in the bottom part. (a) Initially, the two-ion crystal is prepared in the ground state of motion through ground-state cooling (GSC) on the logic ion. (b) Absorption of photons from the pulsed spectroscopy laser results in excitation of motion due to photon-induced recoil. Motional displacements are only in momentum, as the pulses are synchronized with the oscillation period of the normal mode. (c) The motionally excited part of the wavefunction containing Fock states |n>0(represented by the red moon-shaped disc in the phase-space representation) that have no overlap with the ground state |0is converted into an internal-state excitation of the logic ion by a transfer pulse on the red-sideband (RSB). (d) Electron-shelving detection of the internal state of the logic ion provides the spectroscopy signal. Figure 1: Principle of PRS. The top part of the figure shows the internal and motional excitation of the two-ion crystal (spectroscopy (spectr.) ion: top, logic ion: bottom). The centre part shows the Wigner phase-space representation of the excited normal mode. Typical timescales for the experimental implementation are shown in the bottom part. ( a ) Initially, the two-ion crystal is prepared in the ground state of motion through ground-state cooling (GSC) on the logic ion. ( b ) Absorption of photons from the pulsed spectroscopy laser results in excitation of motion due to photon-induced recoil. Motional displacements are only in momentum, as the pulses are synchronized with the oscillation period of the normal mode. ( c ) The motionally excited part of the wavefunction containing Fock states | n >0 (represented by the red moon-shaped disc in the phase-space representation) that have no overlap with the ground state |0 is converted into an internal-state excitation of the logic ion by a transfer pulse on the red-sideband (RSB). ( d ) Electron-shelving detection of the internal state of the logic ion provides the spectroscopy signal. Full size image During interaction with spectroscopy pulses, absorption of a photon displaces the motional state in momentum by ħk , where k is the wavenumber of the spectroscopy light. Efficient excitation of a chosen normal mode is accomplished through application of short (compared with the oscillation period T m in the trap) spectroscopy laser pulses synchronized to the respective normal mode frequency ω m =2 π / T m (refs 26 , 30 , 31 ). The momentum displacement of this mode on absorption of a single photon is given by the Lamb–Dicke factor η (in units of the zero-point momentum fluctuations of the normal mode) [32] . This motional excitation is shared by the logic ion. It is then converted into an electronic excitation of the logic ion via a transfer pulse on the red-sideband. In a simple model, the excitation signal on the logic ion after this pulse is proportional to the probability of leaving the motional ground state, which is approximately given by where N a is the number of absorbed photons. Choosing p e =0.5 yields a SNR of 1 in a single experiment, the best allowed by quantum projection noise [24] . For typical Lamb–Dicke parameters of 0.1, this requires absorption of around 10 photons. An analytical treatment of the observed signal based on a Fokker–Planck equation qualitatively confirms the favourable scaling with the number of absorbed photons and can be found in Supplementary Note 2 . Implementation We have implemented PRS using 25 Mg + as the logic ion to perform an absolute frequency measurement of the 2 S 1/2 ↔ 2 P 1/2 transition in 40 Ca + with a natural linewidth of 21.6 MHz. A sketch of the experimental setup together with the level scheme of the spectroscopy ion is shown in Fig. 2 . Details of the system have been described previously [33] , [34] and are summarized in the Methods section. 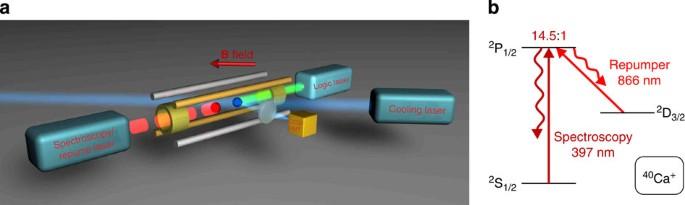Figure 2: Experimental system for photon recoil spectroscopy. (a) Sketch of the experimental setup showing the linear ion trap with spectroscopy ion (red) and logic ion (blue), the laser beam and magnetic field directions, and the detection system for the logic ion. Doppler cooling, detection and sideband manipulation using stimulated Raman transitions are performed on the25Mg+logic ion with light around 280 nm. The two Raman beams are depicted by a single beam corresponding to their relative wave vector Δk. (b) Relevant level scheme for the40Ca+spectroscopy ion. Spectroscopy and repumping on40Ca+require lasers at wavelengths of 397 nm and 866 nm, respectively. The excited2P1/2-state can decay back to the2S1/2or into the long-lived metastable2D3/2state with a branching ratio of 14.5:1. Figure 2: Experimental system for photon recoil spectroscopy. ( a ) Sketch of the experimental setup showing the linear ion trap with spectroscopy ion (red) and logic ion (blue), the laser beam and magnetic field directions, and the detection system for the logic ion. Doppler cooling, detection and sideband manipulation using stimulated Raman transitions are performed on the 25 Mg + logic ion with light around 280 nm. The two Raman beams are depicted by a single beam corresponding to their relative wave vector Δ k . ( b ) Relevant level scheme for the 40 Ca + spectroscopy ion. Spectroscopy and repumping on 40 Ca + require lasers at wavelengths of 397 nm and 866 nm, respectively. The excited 2 P 1/2 -state can decay back to the 2 S 1/2 or into the long-lived metastable 2 D 3/2 state with a branching ratio of 14.5:1. 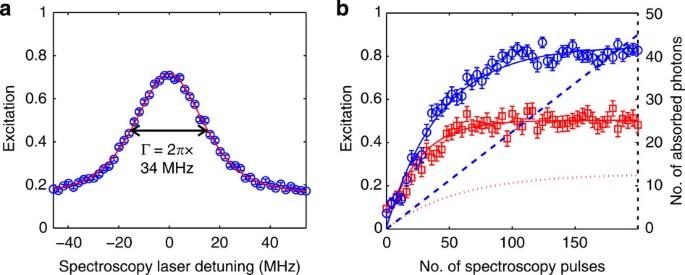Figure 3: Photon recoil spectroscopy results. (a) Frequency scan across the resonance line. The red line is the result of a numerical simulation using calibrated parameters and has been adjusted in amplitude by 0.93 and shifted by 0.15 to account for experimental imperfections (see text for details). (b) On-resonance excitation signal as a function of the number of spectroscopy pulses with (blue circles) and without (red squares) repumper. The solid lines (left axis) are numerical simulations from which the Rabi frequencyΩof the spectroscopy laser is extracted. The dashed and dotted lines (right axis) are derived from the same simulations and give the corresponding integrated number of absorbed photons with and without repumper, respectively. All error bars correspond to 1σstatistical uncertainty. Full size image Resonance line and sensitivity Figure 3a shows the average of 12 scans across the resonance of the 2 S 1/2 ↔ 2 P 1/2 transition in 40 Ca + using PRS as described in Fig. 1 . Typically 70 spectroscopy pulses per cycle are applied and a cycle is repeated 250 times for each frequency point. After each spectroscopy pulse, a repump pulse is applied to clear out the metastable 2 D 3/2 state. The observed linewidth of the transition is ~34 MHz, compatible with Zeeman broadening in the applied bias magnetic field of 5.84(1) × 10 −4 T and Fourier broadening due to the 50-ns short spectroscopy pulses. An additional line broadening due to saturation of the excitation signal for large motional displacements (ground-state depletion) is avoided by choosing a small number of absorbed photons. The line is a numerical simulation of the spectroscopy signal using a full master equation model ( Supplementary Note 3 ) and corrected for experimental imperfections, such as a reduced signal amplitude (typically ≥0.85) from limited sideband transfer efficiency and a signal offset of typically ≤0.15 due to incomplete ground-state cooling. The photon sensitivity of the signal was determined by taking advantage of the excited 2 P 1/2 state branching ratio ( Fig. 2b ). For this, the transition was excited on resonance and the signal amplitudes with and without repumping pulses on 40 Ca + were compared. Figure 3b shows the result as a function of the number of spectroscopy pulses. The Rabi frequency of the spectroscopy laser and the signal per scattered photon is extracted from a numerical simulation of the spectroscopy signal, which takes the excited-state branching ratio of 14.5:1 (ref. 35 ) into account, corresponding to 15.5 absorbed photons in the absence of any repumping. An excitation of p e =0.5 corresponding to SNR=1 in a single experiment is achieved by absorbing 9.5(1.2) photons, in qualitative agreement with equation 1 for our experimental parameters and confirmed by the analytical model ( Supplementary Note 2 ). This high sensitivity even for a small Lamb–Dicke factor of η =0.108 is a consequence of the exponential scaling with the square of the number of absorbed photons (equation 1). Figure 3: Photon recoil spectroscopy results. ( a ) Frequency scan across the resonance line. The red line is the result of a numerical simulation using calibrated parameters and has been adjusted in amplitude by 0.93 and shifted by 0.15 to account for experimental imperfections (see text for details). ( b ) On-resonance excitation signal as a function of the number of spectroscopy pulses with (blue circles) and without (red squares) repumper. The solid lines (left axis) are numerical simulations from which the Rabi frequency Ω of the spectroscopy laser is extracted. The dashed and dotted lines (right axis) are derived from the same simulations and give the corresponding integrated number of absorbed photons with and without repumper, respectively. All error bars correspond to 1 σ statistical uncertainty. Full size image Absolute frequency measurement The main result of this work is shown in Fig. 4 , where we demonstrate that PRS enables precision spectroscopy at an unprecedented level. It shows the results of a frequency measurement of the 2 S 1/2 ↔ 2 P 1/2 transition in 40 Ca + , which we have implemented using a two-point sampling technique [24] . For this, we set the probe laser frequency close to the centre of the atomic resonance and probe the excitation probability for constant frequency steps towards the left and right of the resonance centre. The centre frequency is determined from the average of the excitation probabilities p 1,r on each side, multiplied with the frequency discriminant given by the experimentally determined slope of the resonance curve. These steps are repeated until the desired frequency uncertainty is achieved. The frequency measurements shown in Fig. 4a have been performed on 5 days within 11 weeks. Fig. 4b shows the relative frequency uncertainty as a function of averaging time τ in form of an overlapping Allan deviation σ y ( τ ) (ref. 36 ) of the concatenated five measurement runs. The observed instability σ y ( τ )=5.1 × 10 −9 (red line) is in agreement with the expected Allan deviation of 5.8(9) × 10 −9 given the measured SNR for a single ion using the true measurement time, including dead time from ground-state cooling and detection. This confirms that the measurement is statistics-limited. The required averaging time can be reduced by at least a factor of ten through speed-optimized ground-state cooling [37] . For chosen excitation probabilities p 1,r , the mean number of scattered photons for each probe cycle can be determined from the calibration shown in Fig. 3b . This allows us to express the relative frequency uncertainty as a function of the number N a of absorbed photons, which is given by σ y ( N a )=9.5 × 10 −8 / , corresponding to an uncertainty of 7.2 MHz for 100 absorbed photons. 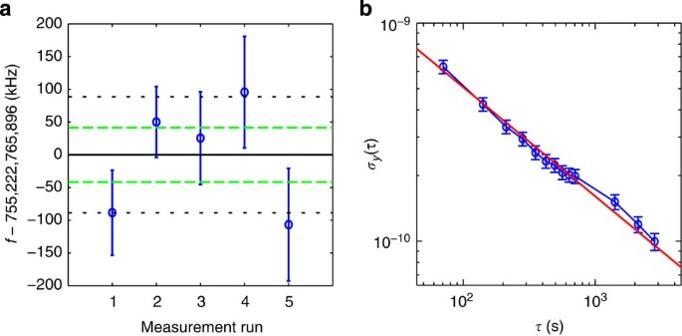Figure 4: Absolute frequency measurement results. (a) Compilation of absolute frequency measurements performed using the two-point sampling technique. The dotted black and dashed green lines give the 68.3% prediction bounds for the measurement and the mean, respectively. (b) Allan deviation of the combined data set. A fit gives an instability ofσy(τ)=5.1 × 10−9. The error bars indicate the s.d. of the mean. Figure 4: Absolute frequency measurement results. ( a ) Compilation of absolute frequency measurements performed using the two-point sampling technique. The dotted black and dashed green lines give the 68.3% prediction bounds for the measurement and the mean, respectively. ( b ) Allan deviation of the combined data set. A fit gives an instability of σ y ( τ )=5.1 × 10 −9 . The error bars indicate the s.d. of the mean. Full size image Table 1 shows a summary of the evaluated systematic effects for the absolute frequency measurement. Details can be found in the Supplementary Notes 1 and 3 . Lineshape asymmetries from an excitation imbalance of Zeeman-shifted line components are strongly suppressed by symmetrical driving of the transition by linearly polarized light. Off-resonant coupling of the spectroscopy laser to other states can cause frequency-dependent AC Stark shifts. We have evaluated both shifts by measuring the line centre frequency as a function of the magnetic field and spectroscopy laser intensity. As expected, the results are compatible with vanishing shifts, limited by the statistical uncertainty of the measurement. Shifts arising from micromotion-induced AC Stark and second-order Doppler effects, as well as lineshape and frequency uncertainties arising from the spectroscopy laser stabilization have been estimated to be well below 1 kHz. The spectral bandwidth of the 125 ns spectroscopy pulses used in the frequency measurements, together with the limited bandwidth of the switching device (an acousto-optical modulator), can cause a shift in the centre frequency of the spectroscopy pulses on the order of ±50 kHz. We calibrate this shift for each experimental run to within 16 kHz. Table 1 Uncertainty evaluation of the absolute frequency measurement. Full size table Probe-frequency-dependent Doppler heating and cooling effects during excitation result in an asymmetric lineshape of the motional excitation signal. Starting from the motional ground state in our system, we have a precise knowledge of the Doppler-induced shifts through the excitation signal. This allows an accurate analytical and numerical calculation of the shift. From a simple model taking into account Doppler-induced (anti)damping and associated narrowing (spread) of the wave packet in momentum space, this frequency shift is given by where we have substituted equation 1 for p 1,r in the last step. The shift increases for smaller excitation probabilities p 1,r used in the two-point sampling technique, corresponding to a larger detuning of the two probe frequencies from resonance and a smaller number of scattered photons. It is worthwhile noting that within the approximations of the model, this shift is independent of the choice of other parameters, such as spectroscopy laser Rabi frequency or the transition linewidth. The result from this simple model agrees very well for typical excitation probabilities between 0.1 and 0.9 with analytical and numerical models including diffusion and drift in position ( Supplementary Notes 2 and 3 ). For smaller excitation probability, the shift is bounded by the trap frequency. From conservatively estimated fluctuations of the detection signal of ±0.1 around p 1,r =0.5, we account for a shift of 151(20) kHz. The uncertainty of this residual Doppler shift can be significantly reduced, while at the same time improving the photon sensitivity, by lowering the trap frequency during spectroscopy. A similar, but much stronger effect from heating/cooling processes during spectroscopy of Doppler-cooled ions has been reduced by sympathetic cooling [38] and interleaved cooling/spectroscopy pulses [20] . The absolute frequency averaged over five individual measurements is 755,222,765,896(88) kHz, of which 78 kHz are from systematic and 42 kHz from statistical uncertainty, in agreement with a previous measurement [20] , but with an accuracy improved by more than an order of magnitude. To our knowledge, this result represents the most accurate absolute frequency measurement of a broad transition in a trapped ion system, resolving the line centre by a factor of more than 300 of the transition’s observed linewidth [7] , [20] , [38] . The high photon sensitivity and absolute frequency accuracy of PRS together with its simplicity, requiring only ground-state cooling, enables spectroscopy of atomic and molecular species inaccessible with other techniques. The method is particularly well suited for systems with non-closed transitions or intrinsically low fluorescence rates, such as molecular ions [39] , [40] , [41] , astro-physically relevant metal ions with a complex level structure [3] , [4] , [42] and highly charged ions [43] . PRS is also an efficient replacement for the original QLS implementation for long-lived excited states, as it does not require the driving of sideband transitions on the spectroscopy ion, thus lowering the requirements on the spectroscopy laser. Combined with the single-photon sensitivity for high photon energies and the background-free detection, PRS enables direct frequency comb [44] , [45] , XUV [46] , [47] and X-ray spectroscopy, [48] , [49] which offer only a small number of photons per spectral bandwidth. This will pave the way for spectroscopic applications ranging from chemistry to fundamental questions in atomic, molecular and nuclear physics. Experimental methods We trap a two-ion crystal consisting of 25 Mg + and 40 Ca + in a linear ion trap at single- 25 Mg + radial and axial trap frequencies of ~5 MHz and 2.22 MHz, respectively. Using resolved sideband cooling [33] on 25 Mg + , we cool the in-phase (ip) and out-of-phase (op) axial modes with frequencies f ip =1.92 MHz and f op =3.51 MHz to their ground state of motion with a typical residual mean occupation of ≈0.07 and ≈0.02. We have chosen the ip-mode as the spectroscopy mode, as it has the largest Lamb–Dicke parameter of = η =0.108 for the calcium ion. The RSB pulse on the logic ion is implemented by a stimulated Raman transition that is red detuned from the | F =3, m F =3 =|↓ ↔|↑ = | F =2, m F =2 transition in the 2 S 1/2 state ( Fig. 5 ) by the normal mode frequency. As the required π -time for optimum transfer depends on the initial motional state [27] , we employ a stimulated Raman adiabatic passage (STIRAP)-like pulse by linearly ramping down the π -Raman beam intensity during 100 μs, while ramping up the intensity of the σ-Raman beam. Although not fully adiabatic, we achieve a more than 80% transfer efficiency of all motionally excited states from |↓ to |↑ , independent of their initial state. Internal state discrimination is performed by applying light resonant with the cycling transition |↓ →| e =| 2 P 3/2 , F =4, m F =4› ( Fig. 5 ) using the π -detection technique [34] . 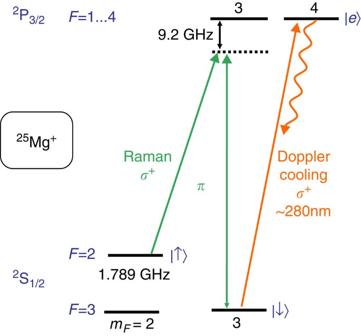Figure 5: Relevant energy levels and transitions in the magnesium logic ion. Ground-state cooling and coherent manipulation are implemented through Raman beams (detuned by 9.2 GHz from the excited state), which couple the two qubit states |F=3,mF=3=|↓, |F=2,mF=2=|↑usingπ- andσ-polarized light. Laser cooling and internal-state discrimination is performed using resonant light with the |↓↔|F=4,mF=4=|eexcited state. Figure 5: Relevant energy levels and transitions in the magnesium logic ion. Ground-state cooling and coherent manipulation are implemented through Raman beams (detuned by 9.2 GHz from the excited state), which couple the two qubit states | F =3, m F =3 =|↓ , | F =2, m F =2 =|↑ using π - and σ -polarized light. Laser cooling and internal-state discrimination is performed using resonant light with the |↓ ↔| F =4, m F =4 =| e excited state. Full size image The 397-nm spectroscopy laser consists of a frequency-doubled extended cavity diode laser. The laser light can be frequency tuned via a double-pass acousto-optical modulator (AOM). An additional AOM is used to provide short (50…125 ns) pulses of spectroscopy light. The intensity-stabilized light is delivered to the atom via a single-mode optical fibre to avoid beam-steering errors. The laser is phase-locked to an optical frequency comb, which is referenced to one of the hydrogen masers at the German National Metrology Institute (PTB), providing a direct link to the SI second (PTB) with a relative frequency uncertainty of better than 10 −12 for averaging times of ~1 h. The spectroscopy and repump light are linearly polarized in a plane spanned by the magnetic field and the trap axis. Under ideal conditions, this results in equal amounts of σ + and σ − polarized light and an additional π component, providing a symmetric spectrum, independent of the magnetic field. Frequency measurements For the final frequency measurement, we employ the two-point sampling method [24] , where the spectroscopy laser probes the excitation signal at the two frequencies ( v 1 = v probe −Δ v FWHM /2, v r = v probe +Δ v FWHM /2), which ideally provides an excitation of half the maximum excitation. In every single scan, the experiment is repeated on both frequencies for 5 × 250=1,250 times. To reduce the detection error, we employ the π -detection method [34] with threshold at 0.5 to extract the excitation probability. This detection scheme is based on post-selection, which inherently reduces the effective number of cycles to a typical value of =1,039(12). This corresponds to a quantum projection noise of σ ( p ) = ≈0.0155. The difference of excitation at the two probe frequencies δ p = p ( v 1 )− p ( v r )= p 1 − p r is used as an error signal to steer the probe frequency v probe towards the line centre in the following scan. The uncertainty for the quantity δ p rescales to σ ( δp ) = ≈0.0220. The excitation difference δp is turned into an absolute frequency v by the following relation where the frequency discriminant D is calibrated for each measurement day experimentally through a measurement of the signal slope around the probe frequencies v 1,r . The final statistical uncertainty for the frequency measurement propagates as where the first term contains the quantum projection noise and the second one the calibration error for the frequency discriminant. Concatenating the time-resolved frequency uncertainty from the five measurements shown in Fig. 4a , the overlapping Allan deviation is derived as shown in Fig. 4b . This gives an inferred instability of 5.1 × 10 −9 for an averaging time of 1 s. This result is in agreement with the quantum projection noise limit of 5.8(9) × 10 −9 estimated according to where T (=70.5 s) refers to the time for repeating the experimental cycles 1250 times. The data shown in Fig. 4 are based on a selection of data that have passed statistical tests to check its validity. A total of seven measurement runs, each performed on a different day, have passed normality tests (Kolmogorov–Smirnov test, Lillifors test, Jarque–Bera test, Shapiro–Wilk test). In a second step, two-sample tests (two-sample Kolmogorov–Smirnov test, two-sample t -test) were performed on every combination of two measurements to verify that all the measurements come from the same normal distribution. Two of them did not pass these tests and were excluded from Fig. 4 . We suspect that the data was contaminated by drifts in the experimental parameters, such as STIRAP and ground-state cooling efficiency, and calibration of the pulse spectrum. After excluding the data that fail the distribution tests, the weighted average of all the frequencies measured on a single day is computed according to with the weight factor w ( i ) =1/( ) 2 . The variance of the mean equals with N as the number of scans on that measurement day. A weighted fit of the centre frequencies from different measurement days with the weights 1/ as in Fig. 4a gives the centre frequency v =755, 222, 765, 896 kHz with a statistical uncertainty of 42 kHz. How to cite this article: Wan, Y. et al. Precision spectroscopy by photon-recoil signal amplification. Nat. Commun. 5:3096 doi: 10.1038/ncomms4096 (2014).